Dynamic protein conformations preferentially drive energy transfer along the active chain of the photosystem II reaction centre One longstanding puzzle concerning photosystem II, a core component of photosynthesis, is that only one of the two symmetric branches in its reaction centre is active in electron transfer. To investigate the effect of the photosystem II environment on the preferential selection of the energy transfer pathway (a prerequisite for electron transfer), we have constructed an exciton model via extensive molecular dynamics simulations and quantum mechanics/molecular mechanics calculations based on a recent X-ray structure. Our results suggest that it is essential to take into account an ensemble of protein conformations to accurately compute the site energies. We identify the cofactor CLA606 of active chain as the most probable site for the energy excitation. We further pinpoint a number of charged protein residues that collectively lower the CLA606 site energy. Our work provides insights into the understanding of molecular mechanisms of the core machinery of the green-plant photosynthesis. Photosynthesis provides the foundation for life by converting sunlight into biochemical energy. By catalysing the oxidation of water to molecular oxygen, the photosystem II (PSII) is a crucial component for photosynthesis [1] , [2] . The PSII is a membrane-bound protein–cofactor complex that contains the antenna complex and reaction centre (RC). Sunlight is first captured by the antenna system and then the excitation energy is trapped in the PSII RC, leading to charge separation and electron transfer with the aid of cofactors, and finally resulting in the production of molecular oxygen [3] , [4] , [5] , [6] . A fascinating fact concerning the PSII is that cofactors are arranged in two branches with a C2 symmetry, but half of them (one complete branch) are not involved in the primary electron transfer from water to plastoquinone [7] , [8] , [9] . Due to this, the underlying C2 branches are termed: active and inactive chains, according to their contributions to the primary electron transfer. Starting from a pair of chlorophyll a (CLA) molecules, each branch contains in order: one accessory CLA, one pheophytin (PHO) and one plastoquinone-9 (PL9). A bicarbonate ion (BCT) coordinated with one non-haem iron is located at the top of the branches. Recently, it has been suggested that the existence of duplicate cofactors in the inactive chain is not superfluous, but to protect the RC from photodamage under high light intensity [10] , [11] . This protection mechanism is achieved by a low quantum yield electron loop with the help of nearby cytochrome b 559 and β-carotene (BCR) [10] , [11] . Understanding how the excitation energy is trapped and transferred in the PSII RC is an essential prerequisite to understand the subsequent preferential electron transfer pathway. Extensive experimental and theoretical studies have attempted to identify the underlying functional states during these processes [7] , [12] , [13] , [14] , [15] , [16] , [17] , [18] , [19] , [20] , [21] , [22] , [23] , [24] , [25] , [26] , [27] , [28] , [29] . Optical spectroscopy is a powerful tool to study the electron and energy transfer processes. However, for PSII, the optical bands of different cofactors are largely overlapped [12] , [13] , [14] , [15] . To overcome this problem, researchers have employed low-temperature optical difference spectroscopy and site-directed mutagenesis of amino acids surrounding the cofactors [30] , [31] , [32] . For example, a mutation of D1-Thr179 (the amino acid spatially close to CLA606) by glutamic acid (Glu) causes a noticeable blue shift (~\n1 nm) in the difference spectrum [32] . Such experiments have shown that CLA606 has a significant contribution to the absorption spectrum, and further suggested that it is the most probable site for the triplet state and local excitation [31] , [32] . Theoretical studies of the experimental spectra also support this observation by showing that CLA606 has the lowest site energy [7] , [16] , [17] , [18] , [25] (that is, the energy necessary to be excited from the ground state to its first excited state or Q y electronic transition [23] ). Therefore, when external energy flows into the RC, CLA606 would serve as the energy trap, because it has the highest probability to be the first cofactor to be driven to the excited state. While spectroscopy has been effective in identifying the functional states of the RC, it is incapable of explaining at the molecular level why CLA606 is the energy trap instead of its symmetric counterpart CLA607. It has been shown that the protein environment can play an important role in directing energy transfer and the subsequent electron transfer process [5] , [33] , [34] , [35] , [36] , [37] . Therefore, theoretical calculations used to understand the underlying molecular mechanism require an explicit consideration of the PSII complex. X-ray crystallography structures of PSII have provided profound insights about the mechanisms of energy transfer in PSII [38] , [39] , [40] , [41] , [42] , [43] . In particular, a recent high-resolution (1.9 Å) structure displays some structural differences between the active and inactive chains [43] . While CLA606 in the active chain and its counterpart CLA607 in the inactive chain are both axially coordinated with water molecules, the water ligand of CLA606 is further hydrogen bonded to Thr179, but that of CLA607 has no such hydrogen bond. However, it is not clear whether the structural differences are sufficient to explain pathway selection or not. In general, one would like to question whether the static crystal structure alone—without considering the protein ensemble under physiological conditions—would suffice to discern between the active and inactive chains in terms of the electron transfer processes. Previous theoretical studies [44] , [45] involving molecular dynamics (MD) simulations (based on low-resolution crystal structures of PSII) have investigated the influence of protein dynamics on energy transfer within PSII. However, none of them addressed the pathway selection for either the energy or electron transfer processes. In this study, we construct an exciton model based on quantum mechanics/molecular mechanics (QM/MM) calculations [36] , [37] , [46] , [47] , [48] , [49] , [50] to elucidate the PSII environmental effect on the preferential selection of energy transfer pathway. In previous theoretical studies, the site energies were determined by spectrum fittings [7] , [16] , [17] , [18] , [25] , a key difference in this work is that these quantities are calculated via atomic-level evaluations involving an ensemble of protein conformations, which has required MD simulations of a system of ~\n580,000 atoms and extensive QM/MM calculations. We find it is crucial to consider an ensemble of PSII complex conformations to identify the preference of energy excitation along the active chain. In contrast, the static crystal structure alone cannot explain such preference. Furthermore, we observe that CLA606 is the most probable site for the energy excitation at both 300 and 77 K, which is consistent with previous spectroscopy studies [7] , [16] , [17] , [18] , [19] , [25] , [31] , [32] . Finally, we have identified at least seven highly conserved and charged protein residues that collectively are responsible of promoting CLA606 as an energy trap in the PSII RC. Validation of MD simulations The PSII complex (see Fig. 1 ) in our MD simulations is stable from the perspective of various structural analyses. The root mean square deviations (r.m.s.d.) of the protein carbon-α atoms relative to the crystal structure are 1.25 and 0.5 Å for 300 and 77 K, respectively (see Fig. 2a ). Overall, stable conformations are observed for all the cofactors in the PSII complex, including CLA, PHO, PL9, BCR, BCT, haem-b (HEM) and the oxygen-evolving complex (OEC) (see Fig. 2a ). For individual cofactors in the RC at 300 K, the r.m.s.d. is below 1.5 Å, except for CLA610, CLA611 and CLA607, which have slightly larger r.m.s.d. (2.0–3.0 Å) (see Fig. 2a ). The higher flexibility of these three cofactors may be due to their less-compact protein environment, especially in the tail regions (see Fig. 1b for their locations in the RC). At 77 K, all the cofactors in the RC are very stable (with r.m.s.d.<1.0 Å). We perform five independent simulations at both 300 and 77 K and each resulting r.m.s.d. curve reach a plateau after 15 ns ( Supplementary Fig. 1 ). To confirm that the system has reached equilibrium, we extended two 300 K simulations to 100 ns, which confirmed that the r.m.s.d. of protein and cofactors in these 100 ns simulations mostly remain a plateau after 15 ns ( Supplementary Fig. 1a,b and Supplementary Methods ). 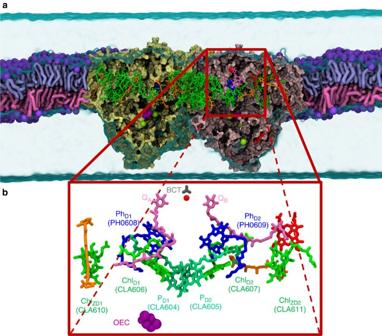Figure 1: The PSII complex and electron transfer chains in its RC. (a) Lateral view of the PSII embedded in the POPC membrane. Our simulation box (254.6 Å × 159.1 Å × 157.7 Å) contains over 578,000 atoms. The two monomers of PSII are shown in yellow and pink. The colour codes for other components are: CLA (green), PHO (blue), PL9 (dark pink), BCR (orange), HEM (red), BCT (grey), non-haem iron (red sphere), OEC (purple spheres) and Cl−(yellow spheres). (b) Cofactors in the electron transfer chains of the RC are coloured and labelled as ina. Figure 1: The PSII complex and electron transfer chains in its RC. ( a ) Lateral view of the PSII embedded in the POPC membrane. Our simulation box (254.6 Å × 159.1 Å × 157.7 Å) contains over 578,000 atoms. The two monomers of PSII are shown in yellow and pink. The colour codes for other components are: CLA (green), PHO (blue), PL9 (dark pink), BCR (orange), HEM (red), BCT (grey), non-haem iron (red sphere), OEC (purple spheres) and Cl − (yellow spheres). ( b ) Cofactors in the electron transfer chains of the RC are coloured and labelled as in a . 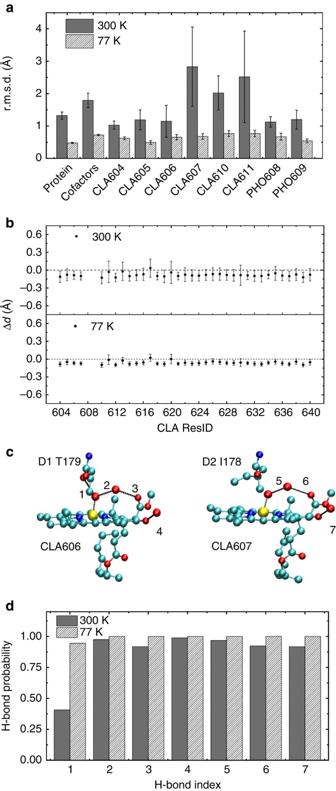Figure 2: MD simulations preserve important protein–cofactor interactions. (a) r.m.s.d. with respect to the crystal structure (PDB ID: 3ARC) for various components of the system are calculated based on MD simulations at 300 and 77 K. The r.m.s.d. of the protein and cofactors (located in the electron transfer chains) are computed based on Cα and heavy atoms, respectively. (b) The deviation from the crystal structure of the distance between the Mg in CLA and its coordinated atom. (c) Hydrogen bonds that CLA606 and CLA607 can form with the protein residues in the crystal structure. (d) The fraction of time that an individual hydrogen bond as shown incis formed in the MD simulations. Full size image Figure 2: MD simulations preserve important protein–cofactor interactions. ( a ) r.m.s.d. with respect to the crystal structure (PDB ID: 3ARC) for various components of the system are calculated based on MD simulations at 300 and 77 K. The r.m.s.d. of the protein and cofactors (located in the electron transfer chains) are computed based on Cα and heavy atoms, respectively. ( b ) The deviation from the crystal structure of the distance between the Mg in CLA and its coordinated atom. ( c ) Hydrogen bonds that CLA606 and CLA607 can form with the protein residues in the crystal structure. ( d ) The fraction of time that an individual hydrogen bond as shown in c is formed in the MD simulations. Full size image Further validations of MD simulations against other properties are based on the conformations from the last 5 ns of those independent 20 ns simulations. The crystal structure of PSII at 1.9 Å resolution (Protein Data Bank (PDB) ID: 3ARC) has identified all axial ligands of CLAs. Seven of them are water molecules and others are amino acids ( Supplementary Table 1 ). In this work, the distance between the Mg atom of each CLA and its coordinated ligand atom evaluated from our MD simulations satisfactorily reproduces that of the crystal structure, with discrepancies being all <0.15 Å (see Fig. 2b ). In the crystal structure, there are four hydrogen bonds around CLA606 and only three around CLA607 (see Fig. 2c ), our MD simulations also reproduce this property (see Fig. 2d ). With the above validations of MD simulations against the crystal structure, we calculated the site energies of cofactors based on our MD conformations to elucidate the molecular mechanism for the unidirectional energy transfer processes. The dynamic environment enables selection of the active chain The C2-symmetric arrangement of cofactors alone cannot explain the pathway selectivity. Therefore, we hypothesized that the dynamics of the PSII environment might play a determinant role in this mechanism. We calculated the site energies of cofactors in the PSII complex with respect to the results in vacuum, using both the static crystal structure and an ensemble of MD conformations (Methods and Supplementary Methods ). 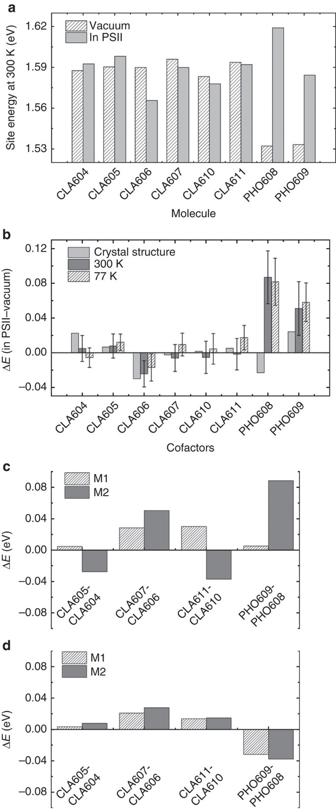Figure 3: PSII complex reduces site energy of the active chain cofactor CLA606. (a) Site energies of the eight cofactors calculated in vacuum and in PSII are compared at 300 K. (b) The site energy shift due to the PSII complex (ΔE=EPSII−Evacuum) are displayed for the static crystal structures (light grey), 300 K MD simulations (dark grey) and 77 K MD simulations (white stripes). (c) Site energy differences between pairs of cofactors located in the active (D1) and inactive (D2) branches are compared for two monomers (M1 and M2) in the crystal structure. (d) The same as inc, except that the results for 300 K MD simulations are shown. Figure 3a reports the calculated site energies of cofactors from the MD conformations of the PSII complex versus those in vacuum at 300 K. While the site energies for CLAs are all comparable in vacuum, the addition of the PSII protein complex allows differentiating them. The site energies of two PHOs, which are substantially lower in vacuum, become comparable with or even higher than those of CLAs in the PSII complex. As shown in Fig. 3b , the effect of PSII complex on the site energies of cofactors in terms of their differences from the vacuum values is comparable at low temperature (77 K) and room temperature (300 K). The most significant effect is observed on CLA606, whose site energy has been greatly reduced by the PSII complex ( Fig. 3a,b , Supplementary Tables 2 and 3 ). The averaged site energy of CLA606 over an ensemble of MD conformations is the lowest one among all the cofactors in the RC. This result is consistent with previous studies [7] , [16] , [17] , [18] , [19] , [25] , where the site energies were obtained by fitting to experimental spectra. In sharp contrast, the PSII complex has nearly zero effect on the site energy of the inactive chain counterpart CLA607. The aforementioned distinct PSII effects on the site energies of these two accessory CLAs differentiate the two chains. Figure 3: PSII complex reduces site energy of the active chain cofactor CLA606. ( a ) Site energies of the eight cofactors calculated in vacuum and in PSII are compared at 300 K. ( b ) The site energy shift due to the PSII complex (Δ E = E PSII − E vacuum ) are displayed for the static crystal structures (light grey), 300 K MD simulations (dark grey) and 77 K MD simulations (white stripes). ( c ) Site energy differences between pairs of cofactors located in the active (D1) and inactive (D2) branches are compared for two monomers (M1 and M2) in the crystal structure. ( d ) The same as in c , except that the results for 300 K MD simulations are shown. Full size image X-ray structure alone fails to explain the pathway preference Figure 3c highlights the fact that the crystal structure alone is insufficient to explain the energy transfer pathway selectivity. In particular, two PSII monomers (M1 and M2) in the crystal structure exhibit inconsistent relative site energies of cofactor pairs. For example, E CLA611 > E CLA610 in M1, while E CLA611 < E CLA610 in M2. The discrepancies between the two monomers are eliminated when an ensemble of conformations are considered (see Fig. 3d ). Thus it is essential to include an ensemble, rather than a single static snapshot, to identify the site energy difference between active and inactive chains. Further comparisons between two chains also show that the site energies of all three CLAs in the active chains are lower than their counterparts in the inactive chain. Among them, the largest difference is between accessory CLA606 and CLA607. We have thus concluded that an ensemble of PSII complex conformations energetically favour the excitation of the cofactors, particularly CLA606 in the active chain over its counterpart in the inactive chain. This further results in a preferential pathway selection for energy excitation of the active chain. The active chain cofactor CLA606 is the energy trap In addition to the excitation of individual cofactor, we construct an exciton model to consider coupling between different cofactors during excitation. Our exciton model shows that the most probable site (30%) for excitation is CLA606 in the active chain at 300 K, indicating that this cofactor serves as an energy trap (see Fig. 4 ). This is in agreement with our previous observation that CLA606 has the lowest site energy among all the RC cofactors. As the temperature decreases from 300 to 77 K, the probability for the energy excitation of CLA606 increases from 30 to 70% ( Fig. 4 and Supplementary Fig. 2 ). This observation is also consistent with previous experimental spectroscopy studies [7] , [16] , [17] , [18] , [19] , [25] , [31] , [32] , which suggested that the excitation probability of CLA606 is 30 and 80% at 300 and 5 K, respectively [19] . Further investigation shows that the decrease in the excitation probability of CLA606 with the increase in the temperature is due to the larger contributions from the high-energy exciton states (see Methods for details). We also find that the effective site energies (and their fluctuations) and coupling strengths at 300 K ( Fig. 4b ) differ from their counterparts at 77 K ( Supplementary Fig. 2b ). This indicates that the effect of protein environment on the excitation of cofactors is temperature dependent and may contribute to the origin of inhomogeneous broadening of the spectrum. 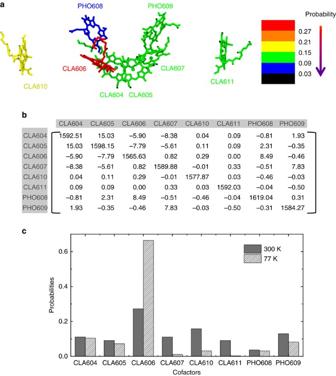Figure 4: CLA606 is the most probable site for the excitation in the RC. (a) Probability of each cofactor in the local excited states at 300 K revealed by the exciton model. The probabilities (Pm) are calculated as weighed sum of each cofactor’s contributions to all the excited states (M) obtained by the exciton model (see equation 2). (b) Exciton matrix (unit: meV) built from 300 K MD simulations. The diagonal terms are the average site energies for the cofactors and the off-diagonal terms correspond to the strengths of the coupling. (c) Comparison between the excitation probabilities of the cofactors at 300 K (dark grey) and those at 77 K (white stripes). Figure 4: CLA606 is the most probable site for the excitation in the RC. ( a ) Probability of each cofactor in the local excited states at 300 K revealed by the exciton model. The probabilities ( P m ) are calculated as weighed sum of each cofactor’s contributions to all the excited states (M) obtained by the exciton model (see equation 2). ( b ) Exciton matrix (unit: meV) built from 300 K MD simulations. The diagonal terms are the average site energies for the cofactors and the off-diagonal terms correspond to the strengths of the coupling. ( c ) Comparison between the excitation probabilities of the cofactors at 300 K (dark grey) and those at 77 K (white stripes). Full size image Protein residues collectively lower CLA606’s site energy As discussed above, we found that the PSII complex is essential for selecting the preferential energy transfer pathway by means of reducing the site energy of CLA606. In this section, we further examine the PSII complex to identify which components have the largest contributions to lower the site energy of CLA606. We studied individually the effects of waters, cofactors and protein components. While the former two have little effect on the site energies, we find that the protein environment reduces the site energy of CLA606 by 0.036 and 0.0 eV at 300 and 77 K respectively, but has almost no effect on CLA607 (see Fig. 5 and Table 1 ). Remarkably, we found that the charged amino acids contribute most to lower the excitation energy of CLA606 (see Table 1 ). We performed single mutant calculations and pinpoint seven critical charged amino acids with each contributing over 0.0035, eV to reducing the site energy of CLA606 (see Fig. 6a,b ). The sole abolition of these amino acids can raise the site energy of CLA606 to almost the same level as its counterpart in the inactive chain CLA607 (see Fig. 6b ). Other charged amino acids have negligible effect. In summary, the seven charged amino acids depicted in Fig. 6 work collectively to lower the excitation energy of CLA606. Interestingly, these charged residues are highly conserved among different species (see Fig. 6c ) and some of them (Glu329, Glu189, Asp170) have been previously identified to have a role in differentiating the cofactor redox potentials of the two chains [51] . Previous site-directed mutagenesis experiments revealed that the mutation of Thr179 to the charged glutamic acid (Glu) leads to a blue shift of ~\n1 nm in the absorption difference spectrum due to the alteration in the excitation energy of CLA606 (refs 31,32) [31] , [32] . Our calculations also show that this mutation can raise the average site energy of CLA606 by ~\n0.005 eV. Even though the absolute site energies have relatively large s.d. (~\n0.02 eV), the shift of the average site energy here may still be meaningful (see Supplementary Methods for the details of mutant calculations). 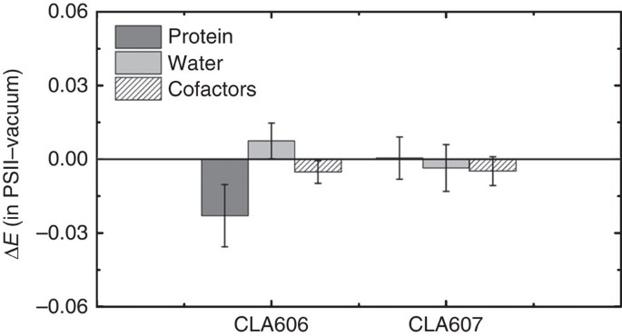Figure 5: The protein plays a crucial role in stabilizing the excitation of CLA606. The effect of protein, waters and cofactors on site energies (ΔE=EPSII−Evacuum) of CLA606 and CLA607 at 300 K are shown in dark grey, light grey and white stripes, respectively. Figure 5: The protein plays a crucial role in stabilizing the excitation of CLA606. The effect of protein, waters and cofactors on site energies (Δ E = E PSII − E vacuum ) of CLA606 and CLA607 at 300 K are shown in dark grey, light grey and white stripes, respectively. Full size image Table 1 The effect of protein residues on site energies of CLA606 and CLA607. 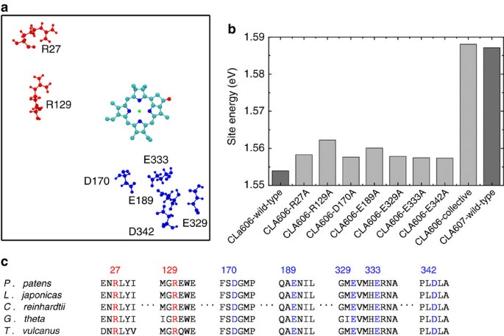Figure 6: Several conserved residues collectively reduce the site energy of CLA606. (a) Charged residues (red: positive-charged; blue: negative-charged) can reduce the site energy of CLA606 over 0.0035, eV individually. The tail of CLA606 is omitted in the figure for clarity. (b) Site energies of CLA606 on seven single mutations are shown. The collective mutations of all these seven residues dramatically increase CLA606’s site energy to almost the same value as its counterpart cofactor (CLA607) in the inactive chain. The wild-type site energies for both CLA606 and CLA607 are also displayed for reference. (c) These seven residues are highly conserved among different species. The sequence alignment was performed with the ClustalW2 program68,69. Full size table Figure 6: Several conserved residues collectively reduce the site energy of CLA606. ( a ) Charged residues (red: positive-charged; blue: negative-charged) can reduce the site energy of CLA606 over 0.0035, eV individually. The tail of CLA606 is omitted in the figure for clarity. ( b ) Site energies of CLA606 on seven single mutations are shown. The collective mutations of all these seven residues dramatically increase CLA606’s site energy to almost the same value as its counterpart cofactor (CLA607) in the inactive chain. The wild-type site energies for both CLA606 and CLA607 are also displayed for reference. ( c ) These seven residues are highly conserved among different species. The sequence alignment was performed with the ClustalW2 program [68] , [69] . Full size image To investigate the effect of the PSII environment on the pathway selection of energy transfer in RC, we have constructed an exciton model ( Fig. 4b and Supplementary Fig. 2b ) on the basis of MD simulations in explicit solvent and extensive QM/MM calculations. From the detailed analysis of the site energy calculations based on the whole PSII complex, we have found that the protein environment determines the difference in probability of energy excitation between the active and inactive chains. In addition, the static protein environment captured by the X-ray crystallography is insufficient to explain the preference of energy excitation along the active chain. It is essential to consider the PSII protein’s structural ensemble to compute accurately the excitation probabilities of its cofactors. We have also observed that CLA606 is the site of energy trap in the PSII complex and may further initiate the charge separation at this site, as has been observed by previous experimental studies [7] , [16] , [17] . Finally, we have identified a small number of charged protein residues in the vicinity of CLA606 collectively lowering its excitation energy. Interestingly, we noticed that the site energies are sensitive to the system complexity. Our simulations and calculations are performed for the whole PSII complex (based on the most detailed crystal structure available), while previously reported experimental spectra were acquired based on minimal scaffold PSII (denoted also as D1-D2-cyt559) [12] , [13] , [14] , [15] , [20] , for which a crystal structure has not yet been reported. Therefore, it is reasonable that some site energy values from our calculations deviate from previous theoretical analysis based on available experimental spectra [11] , [12] , [13] , [23] , [24] , [30] (see the ‘Site energy calculations’ section in Supplementary Methods ). On the basis of these observations, we conclude that CLA606 always has the lowest excitation energy with the presence or absence of the core antenna, while the transition energies of other cofactors are more system-size dependent. Model preparation The crystal structure (PDB ID: 3ARC) at 1.9 Å resolution [40] was used to build up the system for MD simulations. First, we removed the exogenous molecules of diglyceride, alkyl chains, detergents and glycerol. Then, the ‘what if’ suite [52] was used to add the missing lateral chains. The protonation states of His, Asp, Glu, Arg and Lys were automatically determined by Gromacs 4.5 (ref. 53 ). For those His residues in coordination with HEM or CLA, we have manually set their protonation states to maintain the coordination. The PSII complex was inserted into pre-equilibrated lipid bilayers composed of a single-component 1-palmitoyl-2-oleoyl-sn-glycero-3-phosphocholine (POPC) to mimic the natural thylakoid membrane ( Supplementary Methods ). The system was then neutralized by adding 92 sodium ions and solvated in a water box containing 139,935 TIP3P water molecules [54] . Our simulation box (264.3 Å × 165.2 Å × 145.0 Å) contains 578,609 atoms in total (see Fig. 1a ). All-atom AMBER03 force field [55] was chosen for the protein and ions. For the five cofactors (CLA, PHO, BCR, HEM and PL9), force field parameters were previously developed by us [56] . General Amber force field [57] , [58] was adopted for the lipids and bicarbonate, but with a re-fitting of the partial charges following a similar scheme used for the cofactors [56] . The force field parameters for POPC were taken from the previous work by Kasson et al. [59] As suggested by a previous study [44] , we assigned the atomic charges of the OEC complex as follows: Mn1–Mn4, +3; O1–O5, −2; and Ca, +2. To maintain the coordination between the OEC complex and the protein, we have added harmonic restraints with a force constant of 2261.03 kJ mol −1 Å −2 between metal atoms of the OEC and their coordinated protein residues. MD simulations We first performed a 10,000-step energy minimization with the steepest descent algorithm [60] by freezing the PSII complex. The whole system was further energy minimized in another 5,000 steps. Next, the system was simulated with position restrained on all the heavy atoms of the PSII complex with a force constant of 10 kJ mol −1 Å −2 under NVT ensemble ( T =300 K), followed by another 10 ns simulation under NPT ensemble ( T =300 K and P =1 bar). The final configuration from the position-restrained simulation was used to initiate five independent 20 ns production of NPT ( T =300 K and P =1 bar) simulations with temperature annealing from 50 to 300 K in the first 1 ns and different initial velocities (see Supplementary Methods for the simulating parameters). To study the properties at low temperatures, similar procedures and parameters were used to perform another round of MD simulations at 77 K. Following a similar procedure, we also simulated the Thr179Glu mutant ( Supplementary Methods ). All the MD simulations were performed using Gromacs 4.5 (ref. 53 ). Calculation of site energies and coupling strength The Zerner’s Intermediate Neglect of Differential Orbital with parameters for Spectroscopic properties (ZINDO/S) [61] , [62] method (implemented in the ORCA code [63] ) was adopted to calculate the energy gap between the ground state and the first excited state (Q y state) of the cofactor. The last 5 ns of MD simulations was used for the analysis (with a total of 1,250 conformations). For each conformation, we have performed site energy calculation in vacuum, PSII environment and various components of the PSII environment separately (for example, protein, cofactors, waters, charged residues and neutral residues). To account for the environmental effects on the site energy calculations, we have adopted a QM/MM method by treating the cofactors quantum mechanically while the environment as point charges. In particular, we have included atoms within 22 Å of the cofactor and treated them as the point charges ( Supplementary Methods ). In this study, we only considered the excitation to the first excited state (the Q y state) when computing site energies. However, we also note that higher excited states may also play a role depending on the amount of excitation energy transferred to RC from the antenna system. We note that ZINDO/S is a semi-empirical method and the higher-level QM method may be more accurate but also more computationally expensive. To validate the site energies obtained from the ZINDO/S calculations, we also selected representative MD conformations and used higher-level time-dependent density functional theory (LC-wPBE/6-31G(d)) for the site energy calculations. The results from time-dependent density functional theory calculations show reasonable agreement with those obtained from ZINDO/S ( Supplementary Fig. 3 and Supplementary Methods ). To investigate whether the 20 ns simulations have provided a reasonable conformational ensemble for the site energy calculations, we have extended two of the MD simulations at 300 K for 100 ns ( Supplementary Fig. 1a,b ) and used the conformations from the last 5 ns for the calculations. These calculations show similar results to the 20 ns simulations ( Supplementary Fig. 4 ), indicating that the conformations we selected in our site energy calculations within 20 ns represent a reasonable protein structural ensemble (see ‘Site energy calculations’ section in Supplementary Methods for more details). In addition, the appropriated residue protonation states are considered in our site energy calculations ( Supplementary Fig. 5,6 and Supplementary Table 4 ; see `Protonation states of charged residues' section in Supplementary Methods for more details). We have applied the transition charges from electrostatic potentials (TrEsp) method [22] , [64] to determine the coupling strength between pairs of cofactors, in which the transition density of one cofactor was described by the atomic transition charges that were localized at the respective cofactor, and the coupling strength V nm between the two cofactors n and m was given by where indicates the coordinates of the I th atom of cofactor m with the transition charge , while indicates the coordinates of the J th atom of the other cofactor n with the transition charge . f is a distance-dependent factor to account for the solvent effect on the electronic coupling [65] , with f =2.68 × exp(−0.27 × d )+0.54 for two molecules separated by distance d ( Supplementary Fig. 7 and Supplementary Table 5,6 ; see `Coupling strength calculations' section in Supplementary Methods for more details). Exciton model and equilibrium populations The system was described by an effective Hamiltonian, with the diagonal elements describing the site energies of the cofactors and the off-diagonal terms denoting the coupling strength between the cofactors calculated by the TrEsp method [22] , [64] . By diagonalizing the Hamiltonian, the energies of the exciton states were given by the eigenvalues of the Hamiltonian and the components of the corresponding normalized eigenvectors denoted the contributions of each cofactor to the respective exciton state. The probability of excitation on the cofactor m was calculated as: where f (M) is the Boltzmann factor for the exciton state M and is the contribution of the cofactor m to the exciton state M. When the temperature increases, f (M) becomes larger, and exciton states with higher energies will have substantially more contributions to the excitation. Since these exciton states contain a more uniform contribution from various cofactors, it will result in a more flat distribution of excitation probabilities at higher temperature. Sequence alignment We have performed the similarity search of the D1 subunit sequence using the Basic Local Alignment Search Tool (BLAST) program [66] , [67] followed by the multiple sequence alignment by the ClustalW2 program [68] , [69] . How to cite this article: Zhang, L. et al. Dynamic protein conformations preferentially drive energy transfer along active chain of the photosystem II reaction centre. Nat. Commun. 5:4170 doi: 10.1038/ncomms5170 (2014).